Photochemical formation of intricarene Sunlight is the ultimate driver of biosynthesis but photochemical steps late in biosynthetic pathways are very rare. They appear to play a role in the formation of certain furanocembranoids isolated from Caribbean corals. One of these compounds, intricarene, has been suspected to arise from an intramolecular 1,3-dipolar cycloaddition involving an oxidopyrylium. Here we show, by a combination of experiments and theory, that the oxidopyrylium forms under photochemical conditions and that its cycloaddition occurs via a triplet state. The formation of a complex by-product can be rationalized by another photochemical step that involves a conical intersection. Our work raises the question whether intricarene is biosynthesized in the natural habitat of the corals or is an artefact formed during workup. It also demonstrates that the determination of exact irradiation spectra, in combination with quantum chemical calculations, enables the rationalization of complex reaction pathways that involve multiple excited states. Photosynthesis involves the interconversion of light energy into chemical energy, which then drives the complex pathways of secondary metabolism. Photochemical reactions that occur late in a biosynthesis, however, are very rare. In addition, it is often debatable whether they are genuine biosynthetic steps or they take place when biological materials get processed and stored in light. The former seems to apply to the photochemical formation of cholecalciferol (vitamin D 3 ) from 7-dehydrocholesterol. Although the majority of cholecalciferol is taken up from dietary sources, it has been suggested that a lack of sunlight is responsible for the development of rickets and other diseases associated with low levels of vitamin D 3 (ref. 1 ). As with the aetiology of rickets, the geographical latitude and solar irradiance have to be taken into account when the biological significance of photochemical reactions is considered. Situated at the Tropic of Cancer, the Caribbean belongs to the most intensely irradiated regions of the earth. Therefore, it is not surprising that several natural products have been isolated from the Caribbean whose formation seems to require light. The photochemical isomerization of bipinnatin J ( 1 ) to kallolide A ( 2 ) is a case in point ( Fig. 1 ) [2] . Both furanocembranoids have been isolated from gorgonian octocorals, which live at various depths (1–45 m) in the Caribbean Sea and can get exposed to relatively intense sunlight [2] , [3] . It is therefore conceivable that this photochemical reaction, which can be reproduced in high yield in the laboratory [2] , [4] , also occurs in the native environment of the animals. 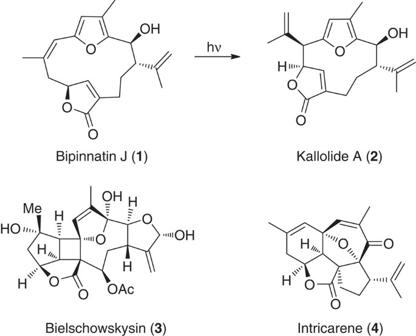Figure 1: Photochemically formed natural products. The natural products relevant to the present work are shown. Figure 1: Photochemically formed natural products. The natural products relevant to the present work are shown. Full size image Bielschowskysin ( 3 ) (ref. 5 ) and intricarene ( 4 ) (ref. 6 ), both isolated from the octocoral Pseudopterogorgia kallos, are two other natural products that have attracted much interest by the synthetic community [7] , [8] , [9] , [10] , [11] , [12] , [13] , [14] , [15] . According to a biosynthetic hypothesis that has been explored by biomimetic total synthesis, intricarene appears to stem from bipinnatin J ( 1 ) as well ( Fig. 2 (refs 7 , 8 )). Oxidation of 1 with photochemically generated singlet oxygen, followed by hydrolysis and rearrangement would yield hydroxy pyrenone 5 . A formal 1,3-elimination of water would then produce an oxidopyrylium 6 , whose diastereoselective transannular 1,3-dipolar cycloaddition would afford intricarene ( 4 ) in a final, concerted step. As such, intricarene could be one of the few natural products whose biosynthesis involves a 1,3-dipolar cycloaddition. 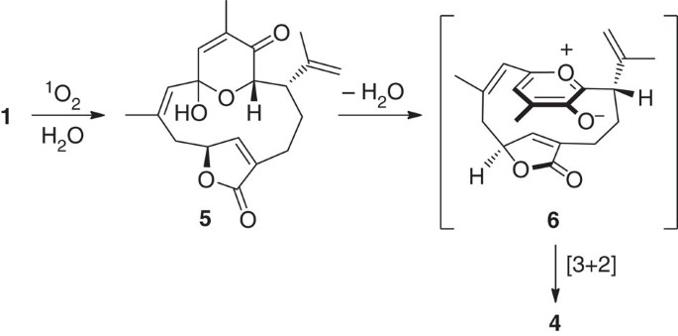Figure 2: Biosynthetic relationship of bipinnatin J and intricarene. Achmatowizc-type oxidation of bipinnatin J, followed by dehydration and 1,3-dipolar cycloaddition was proposed to account for the formation of intricarene. Figure 2: Biosynthetic relationship of bipinnatin J and intricarene. Achmatowizc-type oxidation of bipinnatin J, followed by dehydration and 1,3-dipolar cycloaddition was proposed to account for the formation of intricarene. Full size image Tantillo et al . [16] have provided computational evidence that the key cycloaddition step is thermally feasible. According to their report, however, the calculated activation barrier of ~20 kcal mol −1 (both in nonpolar and polar environments) appears to be relatively high, albeit still within the bounds of a reasonably fast thermal process. Reflecting this value, the published syntheses of intricarene require temperatures and conditions that certainly cannot be deemed ‘biomimetic’ (refluxing DMSO or DMF) and the yields obtained were generally poor [7] , [8] . In addition to this, the exact biosynthetic pathway that would lead from the Achmatowicz oxidation product 5 to the high-energy oxidopyrylium 6 remained unclear. We now show that intricarene can be formed photochemically from a derivative of bipinnatin J ( 1 ) under conditions that resemble those found in the Caribbean. In the course of our studies, we have identified a structurally intriguing by-product that may well be found in extracts from P. bipinnata too. To interpret our results, we have carried out ab initio calculations on the photochemical formation of the oxidopyrylium species and their reactions in the excited state that provide new insights into the chemistry of these useful intermediates. Photochemical synthesis of intricarene Our experimental results were obtained serendipitously during a model study directed at bielschowskysin, the formation of which could also involve photochemistry ( Fig. 3 and Supplementary Discussion ). Treatment of racemic bipinnatin J ( 1 ), obtained by total synthesis [17] , with methanol under slightly acidic conditions gave O -Methyl bipinnatin J ( 7 ). The latter has been isolated before, in enantiomerically pure form, from a methanolic extract of Pseudopterogorgia bipinnata [18] . Oxidation of 7 with singlet oxygen yielded the sensitive diene dione 8 , which, being an ether, cannot undergo acetal formation. Structurally, it resembles the known diene-dione natural products coralloidolide E and isoepilophodione B [19] , [20] . We reasoned that conjugate attack of a molecule of water at C8 of 8 could give rise to enol acetal 9 , which bears the requisite functional groups for a photochemical [2+2] cycloaddition. If successful, this reaction would yield cyclobutane derivative 10 , a close congener of bielschowskysin. 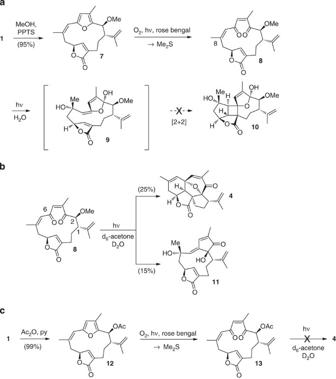Figure 3: Overview of the synthetic route from bipinnatin J (1) to intricarene (4) and hydroxy cyclopentenone 11. (a) Attempted synthesis of the bielschowskysin skeleton via conjugate addition of water and photochemical interception of the presumed intermediate. Conversion of bipinnatin J (1) to its methyl ether8via SN1 reaction was followed by oxidative cleavage of the furan ring to yield diene dione8. Conjugate addition of water was supposed to yield9and enable a photochemical [2+2] cycloaddition to form the central four-membered ring of bielschowskysin. (b) Unexpected formation of intricarene (4) and hydroxy cyclopentenone11under photochemical conditions. (c) Synthesis of acetate12and diene-dione13and failure to yield intricarene under identical photochemical conditions. Figure 3: Overview of the synthetic route from bipinnatin J (1) to intricarene (4) and hydroxy cyclopentenone 11. ( a ) Attempted synthesis of the bielschowskysin skeleton via conjugate addition of water and photochemical interception of the presumed intermediate. Conversion of bipinnatin J ( 1 ) to its methyl ether 8 via S N 1 reaction was followed by oxidative cleavage of the furan ring to yield diene dione 8 . Conjugate addition of water was supposed to yield 9 and enable a photochemical [2+2] cycloaddition to form the central four-membered ring of bielschowskysin. ( b ) Unexpected formation of intricarene ( 4 ) and hydroxy cyclopentenone 11 under photochemical conditions. ( c ) Synthesis of acetate 12 and diene-dione 13 and failure to yield intricarene under identical photochemical conditions. Full size image To mimic Caribbean sunlight, we decided to use a reptile lamp, a type of light source that is known for its significant UV content. Irradiation of 8 in a 1:1 mixture of deuterated acetone and water with a commercially available reptile lamp (nominal power consumption of 275 W) yielded two isolable products. To our considerable surprise, one of them was intricarene ( 4 ), isolated with a yield of 25%, whereas the other one was hydroxy cyclopentenone 11 , which was isolated with a yield of 15%. The X-ray structures of racemic compounds 4 and 11 are shown in Fig. 4 . Structural data of racemic 4 and 11 have been deposited with the Cambridge Crystallographic Data Centre (CCDC accession numbers 1026998 and 1026997, respectively). The photochemical procedure was highly reproducible provided the reptile lamp was used. Notably, it failed when other substrates, such as acetal 5 and acetate 13 , were employed. 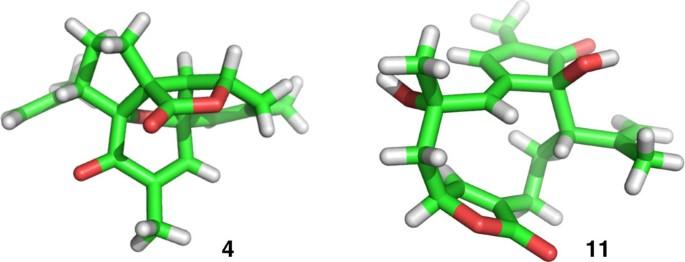Figure 4: X-ray structures of the final products. X-ray structure of racemic intricarene (4) and hydroxy cyclopentenone11. Figure 4: X-ray structures of the final products. X-ray structure of racemic intricarene ( 4 ) and hydroxy cyclopentenone 11 . Full size image Identification of the photo-induced reaction path Our experimental results raise interesting mechanistic and biosynthetic questions, which we decided to address with photophysical considerations and quantum chemical calculations at the CASSCF/CASPT2 and DFT/TDDFT level of theory [21] . Solvation effects (water) were incorporated implicitly by single-point calculations of the optimized gas phase geometries using the state-specific polarizable continuum model (PCM, see Supplementary Table 4 ). As intersystem crossing plays a key role in photochemistry [22] , [23] and intermediate triplet states can be involved in light-induced cycloadditions [24] , [25] , we investigated the singlet as well as the triplet states of the initially excited 8 . As a first step, we measured the emission spectrum of the reptile lamp to compare it with the calculated and experimentally determined absorption spectrum of our starting materials and postulated key intermediates. As can be seen in Fig. 5 , the lamp spectrum has sharp lines in the visible and UV-A region of the electromagnetic spectrum and only negligible contributions below 360 or above 700 nm. The peak emissions at λ max =366, 405, 436, 492, 546, 578 and 679 nm can all be assigned to Hg emissions. This means that UV-B light is virtually absent in this type of lamp, presumably due to the type of glass used for the outer bulb. To determine the irradiance applied in the photochemical synthesis, we determined the light intensity at a distance of 15 cm in front of the lamp (see Supplementary Discussion ). This geometry corresponds to the synthetic conditions. Standard chemical actinometry proved applicable only to a limited extent due to the high intensity of the lamp and the constrained geometry of the NMR tube used as vessel. It therefore provides only a lower boundary. For comparison photometry was also employed that provides an upper boundary for the irradiance. 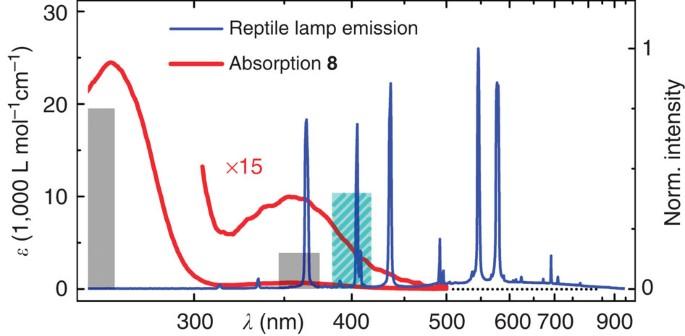Figure 5: Comparison of the precursor absorption spectrum with the illumination spectrum and the calculated transitions. Emission spectrum of the reptile lamp (blue). Absorption of8(red) and calculated transitions for8(grey bars) and6(cyan bar). Figure 5: Comparison of the precursor absorption spectrum with the illumination spectrum and the calculated transitions. Emission spectrum of the reptile lamp (blue). Absorption of 8 (red) and calculated transitions for 8 (grey bars) and 6 (cyan bar). Full size image The experimentally determined absorption spectrum of diene dione 8 shows a weak absorption band in the deep blue and UV-A region around λ max =360 nm and strong absorption around λ max =265 nm ( Fig. 5 ). Only the weak absorption band (360 nm) matches with the emission of our reptile lamp. The photo-initiation of the conversion of 8 therefore has to proceed through the 360 nm transition. In good agreement with the experiment, calculations reveal two absorption bands in the spectral region of interest (grey bars in Fig. 5 ; see Supplementary Methods (quantum chemical calculations) and Supplementary Table 1 and Fig. 3 for details). The most intense band is attributed to an intense ππ* transition from the S 0 to the S 4 state at 260 nm with partial charge transfer character. As the reptile lamp used does not emit in the UV-B region, however, it is irrelevant and we focus on the 360-nm band. For the synthesis the solution of 8 was contained in a standard NMR tube with 4.2 mm inner diameter. We determined the maximum of the molar absorption coefficient of 8 to ε 265 nm=24,500 l mol −1 cm −1 . This renders a value of 670 l mol −1 cm −1 for ε 360 nm and a penetration depth of the UV-A light on the order of 1 mm (see Supplementary Fig. 1 ). As a consequence, certainly all of the light that spectrally overlaps with the 360 nm band (the strong lines at 366, 405 and 436 nm) and penetrates the reaction vessel is absorbed by the bulk sample. The total number of absorbed photons during the 8 h irradiation time is >2 × 10 21 according to the actinometry and <1.2 × 10 22 according to the photometry. This photon number has to be compared with the total of 1.7 × 10 19 molecules of 8 in the 1 ml sample with a concentration of 28 mmol l −1 . Nominally, this means that each molecule would be excited on average >120 times and <700 times. Even if the photochemical quantum yield is as low as 0.01 due to an efficient photophysical return path to the ground state of 8 , practically all molecules will undergo the photochemical conversion in accord with the experimental observation. The long irradiation time ensures that the molecules are sufficiently exchanged by diffusion or most likely convection. Quantum chemical analysis of the reaction path Our rationalization of the photochemical formation of intricarene ( 4 ) and its by-product 11 from diene dione 8 is shown in Fig. 6 . Irradiation of 8 with UV-A light initially populates the excited singlet state 8 (S 1 ). From the quantum chemical calculations, we find that at the Franck-Condon region the S 1 and the T 4 state of 8 are degenerate ( Fig. 6a ). Their spin-orbit coupling has a reasonable size of about 30 cm −1 , consequently effective sub-ps intersystem crossing (ISC) can occur [26] . The resulting excited triplet state 8 (T 4 ) then crosses the transition state TS1(T 1 ), which describes the homolytic bond cleavage of the methoxy group, to yield a triplet diradical 14 (T 1 ). This step corresponds to a photochemical cleavage of an α-carbon-heteroatom bond, a well-known process in carbonyl photochemistry [27] . In case the barrier is not passed and the system relaxes back to the ground state, it can be re-excited and has again the possibility to cross the barrier with a finite probability. The large number of excitation probabilities for each molecule (see above) should allow the system to effectively overcome this barrier. In case no ISC takes place, the system will relax to the S 1 state minimum as high-energy barriers hinder the bond cleavage reaction in the singlet state. In the vicinity of the S 1 minimum a S 1 /S 0 conical intersection seam is reached leading the system again back to the ground state (see Supplementary Table 28 ). 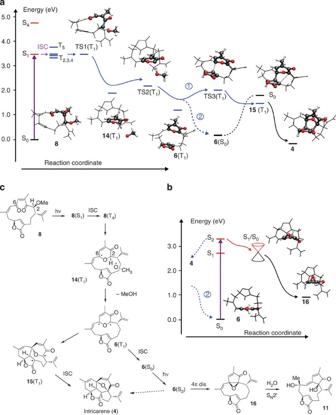Figure 6: Overview of all reactions steps for the proposed mechanism. (a) Calculated reaction path for photo-excited8. Shown are the ΔG values (in eV) for the isolated molecules. Excitation of8with UV-A light and sub-ps ISC to the degenerate T4 state and IC to the T1 state allows the formation of the intermediate diradical14(T1). Next, a hydrogen atom is transferred to afford the triplet diradical6(T1). This intermediate either undergoes a stepwise 1,3 dipolar cycloaddition, including an ISC, to afford4(pathway ), or relaxes to the ground state oxidopyrylium6(S0) (via pathway ). (b) Oxidopyrylium6(S0) can undergo further photochemical reactions. After excitation with blue light to the S2 state, a S1/S0 conical intersection seam can lead to epoxy cyclopentenone16in a reaction that could be interpreted as a conrotatory 4π-electrocyclization. (c) Graphical representation of the reaction path. Vinylogous nucleophilic substitution with water affords11from16. Figure 6: Overview of all reactions steps for the proposed mechanism. ( a ) Calculated reaction path for photo-excited 8 . Shown are the ΔG values (in eV) for the isolated molecules. Excitation of 8 with UV-A light and sub-ps ISC to the degenerate T4 state and IC to the T1 state allows the formation of the intermediate diradical 14 (T 1 ). Next, a hydrogen atom is transferred to afford the triplet diradical 6 (T 1 ). This intermediate either undergoes a stepwise 1,3 dipolar cycloaddition, including an ISC, to afford 4 (pathway ), or relaxes to the ground state oxidopyrylium 6 (S 0 ) (via pathway ). ( b ) Oxidopyrylium 6 (S 0 ) can undergo further photochemical reactions. After excitation with blue light to the S2 state, a S1/S0 conical intersection seam can lead to epoxy cyclopentenone 16 in a reaction that could be interpreted as a conrotatory 4π-electrocyclization. ( c ) Graphical representation of the reaction path. Vinylogous nucleophilic substitution with water affords 11 from 16 . Full size image Once formed, the triplet diradical 14 (T 1 ) undergoes hydrogen transfer via the transition state TS2(T 1 ) to yield triplet oxidopyrylium 6 (T 1 ) and methanol. According to our calculations, the oxidopyrylium 6 (T 1 ) in its triplet state has two possible fates: initial bond formation between C6 and C11, via transition state TS3(T 1 ), yields triplet diradical 15 (T 1 ), which undergoes intersystem crossing and a second bond formation to furnish intricarene ( 4 ) (pathway ). Overall, this amounts to a stepwise cycloaddition. Alternatively, relaxation of 6 (T 1 ) to the oxidopyrylium ground state 6 (S 0 ) can occur (pathway ). The calculated absorption spectrum of 6 (S 0 ) at λ max =405 nm is well-matched with the emission spectrum of the reptile lamp (see Fig. 5 , cyan bar; see Supplementary Table 5 and Fig. 4 for details), allowing it to undergo another photochemical reaction. After excitation to 6 (S 2 ) a low lying conical intersection seam connecting all three singlet states S 2 , S 1 and S 0 can be reached. The geometry leading to the formation of epoxy cyclopentenone 16 is marked as S 1 /S 0 -CoIn in Fig. 6b (see Supplementary Tables 6 and 33 ). From a more synthetic point of view, this process can be classified as a disrotatory electrocyclization in the excited state. From 6 (S 2 ), the formation of intricarene ( 4 ) can also occur via the T 1 state and via conical intersections among the singlet states. In the presence of water, the vinyl epoxy cyclopentenone 16 is presumably highly unstable. We propose that it undergoes vinylogous nucleophilic substitution to afford the experimentally observed hydroxy cyclopentenone 11 . Our mechanism for the formation of the oxidopyrylium via homolytic bond cleavage in the excited state explains why the reaction can take place in the presence of water and why the acetate 13 failed to yield intricarene. The bond dissociation energy (BDE) of methanol ( DH 298 =104.6±0.7 kcal mol −1 ) is significantly lower than that of water ( DH 298 =118.82±0.07 kcal mol −1 ). In contrast, homolytic cleavage of the acetate 13 would yield a highly unstable acetoxy radical (the BDE of acetic acid is DH 298 =112±3 kcal mol −1 ) and is therefore less favourable than the homolytic cleavage of methyl ether 8 (ref. 28 ). Our work raises interesting questions regarding the classification of intricarene as a natural product. We define a natural product as a compound that is present within or in the immediate vicinity of the producing organism. As such, many compounds that are spontaneously formed from reactive intermediates, for instance via cascade reactions [29] , [30] , [31] , [32] , [33] , [34] , can indeed be classified as natural products. Our hypothetical starting material O -Methyl bipinnatin J ( 7 ), however, has been suspected to be an isolation artefact as methanolysis of bipinnatin J ( 1 ) and of kallolide ( 2 ) is a very facile process [18] . In addition, while 4 could biosynthetically formed from 1 and S -adenosyl methionine by an O -methyl transferase, it is conspicuous that 4 is the only C2 methyl ether known in the entire furanocembranoid series [35] . In the course of the isolation of intricarene, P. kallos was partially sun-dried (with indirect sunlight), frozen and lyophilized before extraction [6] . The dry organism was blended using a 1:1 mixture of dichloromethane and methanol. This suggests that the photochemical oxidation and cycloaddition could have taken place during workup. In contrast, clear sea water is known to only weakly attenuate UV-A/blue light [36] , [37] . Thus, at a depth of 25–28 m, where the octocoral was collected, the intensity of incident UV-A and blue light is still well within the range of indirect sunlight at sea level and high enough to promote the proposed photochemistry over time (see Supplementary Fig. 2 and Supplementary Discussion (Irradiance in the natural habitat of the coral)). All things considered, we cannot decide whether intricarene is a genuine natural product according to the definition given above or an isolation artefact that was formed in the course of the isolation/purification procedure. This question could be settled by isolating intricarene under conditions that rigorously exclude air, intense light and methanol during workup. In sum, our work provides a rationale for the formation of intricarene, which is based on photochemistry and overcomes the need to invoke a thermally challenging 1,3-dipolar cycloaddition. Our quantum chemical calculations provide detailed insights into the largely unexplored excited state chemistry of oxidopyrylium species. Finally, our results demonstrate that photochemical reactions, especially reaction cascades that proceed through a series of intermediates, need to be properly matched to the emission spectrum of the lamp used. As absorption spectra of putative intermediates can nowadays be calculated with relative ease, detailed information on the light source will greatly facilitate the planning and execution of photochemical reactions. How to cite this article: Stichnoth, D. et al . Photochemical formation of intricarene. Nat. Commun. 5:5597 doi: 10.1038/ncomms6597 (2014). Accession codes: The X-ray crystallographic coordinates for structures reported in this article have been deposited at the Cambridge Crystallographic Data Centre (CCDC), under deposition numbers CCDC 1026998 and 1026997 . These data can be obtained free of charge from The Cambridge Crystallographic Data Centre via http://www.ccdc.cam.ac.uk/data_request/cif .